Chimeric viruses blur the borders between the major groups of eukaryotic single-stranded DNA viruses Metagenomic studies have uncovered an astonishing diversity of ssDNA viruses encoding replication proteins (Reps) related to those of eukaryotic Circoviridae , Geminiviridae or Nanoviridae ; however, exact evolutionary relationships among these viruses remain obscure. Recently, a unique chimeric virus (CHIV) genome, which has apparently emerged via recombination between ssRNA and ssDNA viruses, has been discovered. Here we report on the assembly of 13 new CHIV genomes recovered from various environments. Our results indicate a single event of capsid protein (CP) gene capture from an RNA virus in the history of this virus group. The domestication of the CP gene was followed by an unprecedented recurrent replacement of the Rep genes in CHIVs with distant counterparts from diverse ssDNA viruses. We suggest that parasitic and symbiotic interactions between unicellular eukaryotes were central for the emergence of CHIVs and that such turbulent evolution was primarily dictated by incongruence between the CP and Rep proteins. Single-stranded (ss) DNA viruses represent a rapidly expanding, diverse supergroup of economically, medically and ecologically important pathogens preying on hosts from all three domains of life. On the basis of genetic and structural properties, they are classified by the International Committee on Taxonomy of Viruses into eight families— Anelloviridae , Bidnaviridae , Circoviridae , Geminiviridae , Inoviridae , Microviridae , Nanoviridae and Parvoviridae [1] —whereas some groups still await proper taxonomical assessment [2] , [3] , [4] . ssDNA viruses infecting plants (geminiviruses and nanoviruses) and animals (anelloviruses, circoviruses and parvoviruses) were in the spotlight of extensive research for many years due to their direct effect on the well-being of humans. Recently, a previously unsuspected facet of the ssDNA viruses as important factors in the global ecosystems has come to light; viruses with ssDNA genomes have been repeatedly isolated from diverse environments, including extreme geothermal [2] and hypersaline habitats [3] , [5] , soil [6] , freshwater and marine ecosystems [7] , [8] , [9] . Whereas some bacterial and archaeal ssDNA viruses display filamentous or pleomorphic (variable appearance) virion morphologies [2] , [3] , [10] , all eukaryotic ones (namely Anelloviridae , Bidnaviridae , Circoviridae , Geminiviridae , Nanoviridae and Parvovriridae ) pack their genomes into small icosahedral capsids, constructed from multiple copies of a single (for example, geminiviruses) or several (for example, parvoviruses) nearly identical capsid proteins (CP) [11] . In all cases when high-resolution structural information is available, the CPs of ssDNA viruses were found to display a jelly-roll (antiparallel eight-stranded β-barrel) fold, which is also found in the vast majority of icosahedral positive-sense ssRNA viruses infecting eukaryotic hosts [12] , [13] . At the sequence level, however, the similarity between the CPs of viruses belonging to different families is not recognizable. Another feature that is common to eukaryotic ssDNA viruses is the mechanism of genome replication; the vast majority of these viruses are believed to replicate their genomes via the rolling-circle (RC) or catalytically similar rolling-hairpin mechanism mediated by homologous virus-encoded RC replication initiation proteins (RC-Rep) [13] , [14] . In this respect, ssDNA viruses resemble prokaryotic RC plasmids, pointing towards a possible evolutionary link between these two types of mobile genetic elements [13] , [14] , [15] . A characteristic feature of RC-Reps of eukaryotic ssDNA viruses is the presence of the superfamily 3 helicase (S3H) domain [16] , [17] , which is fused carboxy-terminally to the catalytic nuclease domain encompassing three signature motifs found in all prokaryotic and eukaryotic virus and plasmid RC-Reps [14] . As opposed to CPs, RC-Reps of eukaryotic viruses display actual sequence similarity and RC-Rep-based phylogenies recapitulate the major taxonomic groups defined by the International Committee on Taxonomy of Viruses [1] , [18] , [19] . However, it should be noted that not all eukaryotic ssDNA viruses possess genes for canonical RC-Reps; for example, anelloviruses—even though believed to replicate via RC mechanism—do not encode a protein that would contain the entire set of motifs characteristic to RC-Reps [17] . The origin(s) and evolutionary relationships between ssDNA viruses belonging to different families remain obscure. Structural similarity between the CPs of bacterial microviruses and eukaryotic parvoviruses, circoviruses and geminiviruses [11] was suggested to testify for the common origin of these viruses [20] . Alternatively, similarity between the RC-Reps of ssDNA viruses and prokaryotic plasmids on the one hand [14] , [15] , [21] , [22] and structural similarity between the CPs of viruses with ssDNA and ssRNA genomes on the other [13] led to the proposal that different groups of ssDNA viruses have emerged from plasmids by acquisition of CP-coding genes from RNA viruses, possibly on multiple independent occasions [12] , [13] , [23] . Indeed, both homologous and illegitimate recombination have important roles in driving the evolution of ssDNA viruses [19] . During the past few years, numerous studies on uncultivated viral communities using metagenomic approaches have revealed that genetic diversity of ssDNA viruses is much greater than originally recognized (reviewed in refs 17 , 18 ). Many of these uncultivated viruses are related to members of the bacteriophage family Microviridae [9] , but perhaps even larger number encode RC-Reps displaying phylogenetic affinity to one of three families of eukaryotic ssDNA viruses— Circoviridae , Geminiviridae and Nanoviridae (for example, see refs 24 , 25 , 26 , 27 ). Interestingly, instead of encoding genes for corresponding CPs (circo-, gemini- and nano-like), these viruses typically bear open-reading frames that do not share appreciable similarity with sequences in the databases. Potentially, the lack of recognizable sequence similarity might be caused by the extremely high mutation rates characteristic to ssDNA viruses [28] , [29] . Thus, to navigate in the constantly increasing pool of environmental viral genomes, RC-Reps are often used as markers for classification of the uncultivated ssDNA viruses. Recently, Diemer and Stedman [30] have described a novel chimeric viral (CHIV) ssDNA genome recovered from a hot, acidic Boiling Springs Lake (BSL), USA. Whereas the RC-Rep of the virus was most similar to those of circoviruses, the CP was highly similar to the CPs of ssRNA viruses of the family Tombusviridae and two unclassified oomycete-infecting viruses, Sclerophthora macrospora virus A (SmV-A) and Plasmopara halstedii virus A (PhV-A) [30] . Notably, the tombusvirus-like CP topology has not been previously observed for any DNA virus, suggesting that the virus has emerged via recombination between a DNA and an RNA virus [31] . The validity of the assembled viral genome, tentatively named the RNA–DNA hybrid virus (BSL_RDHV), and its presence in the lake sediment pore water were confirmed by PCR amplification [30] . Importantly, the finding that RNA and DNA viruses recombine to produce novel chimeric entities rationalizes some of the puzzles of the virosphere and allows assessing new hypotheses on the origin and evolution of different viral groups [12] , [13] . Here we report on the assembly of 13 new CHIV genomes recovered from various environments, and encoding tombusvirus-like CPs and, unexpectedly, diverse RC-Reps related to the corresponding proteins of eukaryotic ssDNA viruses belonging to three different families. We show that the history of this virus group involved a unique event of CP gene capture from an RNA virus, followed by an unprecedented recurrent replacement of the Rep genes in CHIVs with distant counterparts from diverse ssDNA viruses. Frequent exchange of Rep genes described here blurs the borders between the major groups of eukaryotic ssDNA viruses and suggests that Reps represent an inadequate marker for tracing their evolutionary history. Finally, we suggest that parasitic and symbiotic interactions between unicellular eukaryotes were central for the emergence of CHIVs. New CHIVs To get further insight into the diversity and evolution of CHIVs, we have assembled sequence reads from 103 publicly available viromes and searched the resultant contigs for co-occurrence of genes encoding RC-Reps and RNA virus-like CPs ( Supplementary Data 1 ). As a result, nine contigs were assembled from viromes derived from atmospheric [32] and aquatic [26] , [33] , [34] samples. As ssDNA viruses are known to integrate into the genomes of their hosts [35] , [36] , we also searched for the presence of CHIVs in the eukaryotic genome databases. The latter approach yielded four additional contigs matching our criteria. Three of these represented contigs from two different whole-genome shotgun (WGS) libraries of marine photosynthetic picoeukaryote populations dominated by the green alga Bathycoccus [37] , whereas the fourth one was from a WGS library of Astrammina rara , a foraminiferan protist [38] . General characteristics of the 13 CHIV genomes (CHIV1–13) obtained by the two approaches are summarized in Fig. 1 and Supplementary Data 2 . In accordance with the experimentally verified topology of the BSL_RDHV genome [30] , most (9 out of 13) of the CHIV contigs obtained here are circular. Importantly, the potential stem loops containing nonanucleotide sequences, which serve as origins of replication in ssDNA viruses with circular genomes [17] , are readily identifiable in proximity of the RC-Rep genes in all CHIV genomes ( Supplementary Data 2 and Fig. 1 ). Besides the CP and RC-Rep genes, some of the CHIVs are predicted to contain up to four additional open-reading frames. However, sequence analysis does not offer any insight into their possible functions. 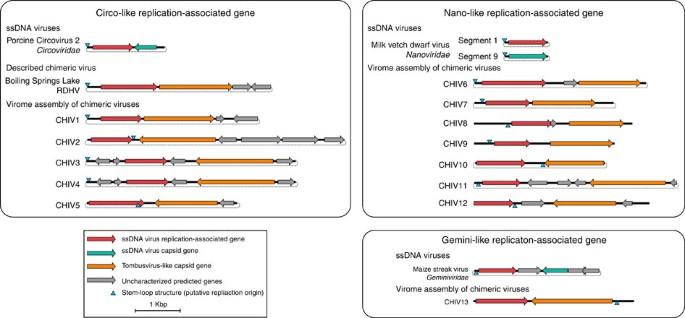Figure 1: Genomic maps of CHIVs and representative reference genomes. CHIVs are grouped according to the type of Rep they encode. Arrows denote open-reading frames. The colour key is provided in the figure. The location and orientation of the potential stem loops containing nonanucleotide motifs are indicated with light blue triangles. CHIV13 genome is reverse-complemented for more convenient representation. Figure 1: Genomic maps of CHIVs and representative reference genomes. CHIVs are grouped according to the type of Rep they encode. Arrows denote open-reading frames. The colour key is provided in the figure. The location and orientation of the potential stem loops containing nonanucleotide motifs are indicated with light blue triangles. CHIV13 genome is reverse-complemented for more convenient representation. Full size image Emergence of CHIVs is a rare event All CHIVs encode putative CPs related to those of tombusviruses, to the exclusion of all other groups of RNA viruses. We note that recent exploration of the ssDNA virus diversity associated with dragonflies revealed a viral genome, DfCyclV, encoding a putative protein with weak but significant similarity to the CP of satellite tobacco necrosis virus [25] . The authors concluded that DfCyclV might be a CHIV with a circovirus-like RC-Rep and a tombusvirus-like CP. However, the satellite tobacco necrosis virus CP is radically different in sequence and structure from those of tombusviruses and most closely resembles the CPs of geminiviruses [21] . Thus, in our opinion, DfCyclV should not be confused with BSL_RDHV-like CHIVs. Members of the family Tombusviridae have positive-sense ssRNA genomes and infect a variety of land plants [39] , although several tombusviruses have also been isolated from freshwater samples [40] . Viruses belonging to Tombusviridae genera Aureusvirus , Avenavirus , Carmovirus , Dianthovirus and Tombusvirus possess icosahedral virions with a granular surface. The latter property is determined by a unique domain organization of the CPs of these viruses. Each CP subunit consists of three distinct domains: the amino-terminal RNA-binding (R) domain facing the interior of the virion, the shell (S) domain central for the assembly of the icosahedral capsid and the C-terminal projection (P) domain, which faces away from the capsid surface, giving the virion its granular appearance ( Fig. 2a,b ). Outside of the Tombusviridae , the same CP domain organization is expected (based on sequence similarity) only for two recently isolated unclassified oomycete-infecting ssRNA viruses, SmV-A and PhV-A [41] , [42] . 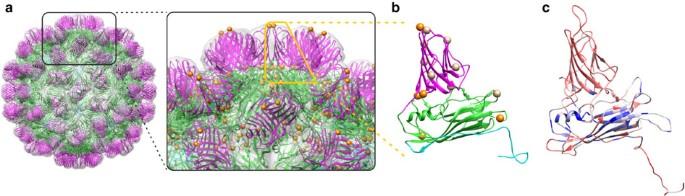Figure 2: Insights into the structure of CHIVs. (a) Structure of the MNSV (PDB ID:2ZAH) is shown to illustrate the contribution of the distinct CP domains to the virion organization and the position of these domains in the capsid surface lattice. The P-domain, magenta; S-domain, green; R-domain, cyan. On the right is a zoom-in on one of the capsid areas, where locations of the conserved insertions present in the CPs of CHIVs, as well as viruses SmV-A and PhV-A are indicated with orange spheres. (b) Structure of the MNSV CP. The P-, S- and R-domains, as well as the locations of conserved insertions are coloured as ina. In addition, the locations of species-specific sequence insertions present in the CPs of only some CHIVs are indicated with grey spheres. (c) Structural model of the CHIV10 CP. The colouring represents sequence conservation among CHIV CPs (red, least conserved; blue, most conserved). Figure 2: Insights into the structure of CHIVs. ( a ) Structure of the MNSV (PDB ID:2ZAH) is shown to illustrate the contribution of the distinct CP domains to the virion organization and the position of these domains in the capsid surface lattice. The P-domain, magenta; S-domain, green; R-domain, cyan. On the right is a zoom-in on one of the capsid areas, where locations of the conserved insertions present in the CPs of CHIVs, as well as viruses SmV-A and PhV-A are indicated with orange spheres. ( b ) Structure of the MNSV CP. The P-, S- and R-domains, as well as the locations of conserved insertions are coloured as in a . In addition, the locations of species-specific sequence insertions present in the CPs of only some CHIVs are indicated with grey spheres. ( c ) Structural model of the CHIV10 CP. The colouring represents sequence conservation among CHIV CPs (red, least conserved; blue, most conserved). Full size image To better understand the relationship between the CPs of ssRNA viruses and CHIVs, we built a three-dimension model of a representative CHIV CP; CHIV10 (Airborne_IC2) was chosen for this purpose ( Fig. 2c ). In accordance with previous predictions [30] , good stereochemical quality of the obtained structural model ( Fig. 3 ) confirms that the CPs of CHIVs are likely to display the same structural fold and domain organization as those of tombusviral CPs. Comparison of the 14 CHIV CPs (13 new and 1 from BSL_RDHV) in the context of their tertiary structures reveals that the most conserved part of these proteins corresponds to the S-domain, whereas the R- and P-domains are much more variable ( Fig. 2c , Supplementary Fig. S1 ). Similar pattern of conservation has been also observed in tombusviruses [43] . Closer examination of the multiple alignment of CHIV, tombusviral and oomycete-infecting virus (SmV-A and PhV-A) CP sequences shows that CHIV CPs are more closely related to the proteins of SmV-A and PhV-A than they are to the CPs of tombusviruses. Five unique insertions, not present in tombusviral CPs, are shared between the CPs of CHIVs, SmV-A/PhV-A and the related sequences from the Lake Needwood RNA virome (indicated with orange spheres in Fig. 2a,b ; see also Supplementary Fig. S1 ), which we consider as synapomorphies testifying for the common evolutionary history of these proteins. Furthermore, unlike in tombusviruses, but similar to that in SmV-A/PhV-A, CHIV capsids are not likely to be stabilized by calcium ions; none of the CHIV CPs contains the calcium-binding motifs, as has been also noted for BSL_RDHV [30] . Finally, eight species-specific insertions are present in the CPs of certain CHIVs (grey spheres in Fig. 2b , see also Supplementary Fig. S1 ). Most of them are located within the P-domains. Importantly, alterations within the P-domain are less likely to interfere with capsid formation, which is primarily orchestrated by interactions within the S-domain. We hypothesize that the P-domain is involved in virus–host interaction (possibly host recognition), which would explain its greater variability promoted by a constant arms race between the virus and the host [44] . 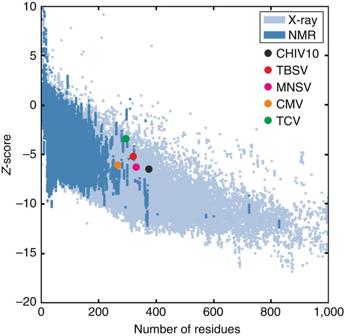Figure 3: Quality assessment of the three-dimensional model of the CHIV10 CP. Quality of the generated model along with that of structural homologues used for modelling (see Methods section) was evaluated using PsoSA-web athttps://prosa.services.came.sbg.ac.at/prosa.php.The calculated quality (Z) scores (closed circles) are displayed in the context of theZ-scores of all experimentally determined protein structures available in the Protein Data Bank. Every dot represents a distinct structure solved by X-ray crystallography (light blue) or NMR (dark blue). TBSV, tomato bushy stunt virus; MNSV, melon necrotic spot virus; CMV, carnation mottle virus; TCV, turnip crinkle virus. Figure 3: Quality assessment of the three-dimensional model of the CHIV10 CP. Quality of the generated model along with that of structural homologues used for modelling (see Methods section) was evaluated using PsoSA-web at https://prosa.services.came.sbg.ac.at/prosa.php. The calculated quality ( Z ) scores (closed circles) are displayed in the context of the Z -scores of all experimentally determined protein structures available in the Protein Data Bank. Every dot represents a distinct structure solved by X-ray crystallography (light blue) or NMR (dark blue). TBSV, tomato bushy stunt virus; MNSV, melon necrotic spot virus; CMV, carnation mottle virus; TCV, turnip crinkle virus. Full size image To learn on how many independent occasions tombusvirus-like CP genes were captured by DNA viruses, we performed a maximum-likelihood phylogenetic analysis of the CHIV, tombusviral and SmV-A/PhV-A CP proteins ( Fig. 4 ). In addition, the data set was supplemented with tombusvirus-like CP sequences recovered from the RNA virome obtained from Lake Needwood [45] . Notably, in none of the data sets containing information about both RNA and DNA virus communities present in the same environmental sample [34] could we detect both CHIVs and tombus-like RNA viruses (in the DNA and RNA fractions, respectively), pointing towards their divergent distribution. The tombusvirus sequences form a well-supported monophyletic clade. Interestingly, all CHIVs cluster together as a sister group to the CPs of SmV-A/PhV-A ( Fig. 4 ). Monophyly of the CHIV CPs and the fact that no other RNA virus-like CPs were found in association with RC-Reps suggest that transfer of a CP gene between RNA and DNA viruses was a unique event and that emergence of CHIVs is likely to be rare. 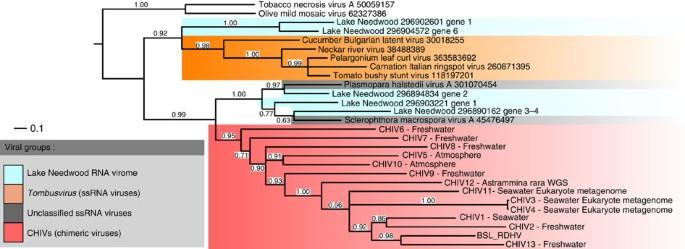Figure 4: Phylogenetic tree of tombusvirus-like CPs. CHIVs are highlighted in red, tombusviruses in orange and unclassified ssRNA viruses are either in grey when isolated, or in blue when assembled from Lake Needwood RNA virome. Tobacco necrosis virus A and Olive mild mosaic virus, both members of the genusNecroviruswithinTombusviridae, have CPs lacking the P-domain and were used as external group. Numbers at the branch points represent SH-like local support values (based on 1,000 resamples), and nodes with scores <0.5 were collapsed. NCBI GI numbers are indicated for all reference sequences. Figure 4: Phylogenetic tree of tombusvirus-like CPs. CHIVs are highlighted in red, tombusviruses in orange and unclassified ssRNA viruses are either in grey when isolated, or in blue when assembled from Lake Needwood RNA virome. Tobacco necrosis virus A and Olive mild mosaic virus, both members of the genus Necrovirus within Tombusviridae , have CPs lacking the P-domain and were used as external group. Numbers at the branch points represent SH-like local support values (based on 1,000 resamples), and nodes with scores <0.5 were collapsed. NCBI GI numbers are indicated for all reference sequences. Full size image Polyphyly of RC-Reps in CHIVs Sequence analysis of CHIV RC-Reps reveals a domain organization typical of eukaryotic ssDNA viruses, with the N-terminal nuclease domain and the C-terminal S3H domain [14] , [17] . The three signature motifs of the nuclease domain are readily identifiable in all CHIV RC-Reps, whereas the S3H motifs are conserved in all but two proteins—Walker B motif could not be mapped in the RC-Reps of CHIV6 and CHIV12 ( Table 1 ). Previous analysis of the RC-Rep encoded by BSL_RDHV showed that it is most closely related to those of circoviruses [30] . Unexpectedly, BLASTp analysis performed in this study reveals differential affinity of the CHIV RC-Reps to the corresponding proteins from three major groups of eukaryotic ssDNA viruses. The latter observation is confirmed by phylogenetic analysis of RC-Reps encoded by CHIVs, circoviruses, nanoviruses and geminiviruses ( Fig. 5 ). Similar to that in the case of BSL_RDHV, five CHIVs (CHIV1–5) cluster with circoviruses. CHIV6–12 form a well-supported phylogenetic clade with nanoviruses, whereas CHIV13 branches together with geminiviruses, separately from the rest of CHIVs ( Fig. 5 ). The significance of a tree topology can be assessed using a constrained tree approach, as demonstrated previously for other viruses [46] . To verify the validity of the obtained grouping of CHIV RC-Reps, the likelihood of the original tree ( Fig. 5 ) was compared with the likelihood of a tree constrained for CHIV monophyly (see Methods section). In this analysis, the monophyly is unequivocally rejected ( Table 2 ) at a statistically significant level ( P -value <0.001), confirming the polyphyly of CHIV RC-Reps. By contrast, the constrained tree strongly enforces the monophyly of CHIV CPs and cannot be rejected by statistical tests ( Table 2 ). Such phylogenetic distribution of CHIV RC-Reps is in stark contrast with the monophyly of the CHIV CPs. Indeed, the CHIV pairs that are close on the CP tree fall into different clades on the RC-Rep phylogeny. For example, the three CHIVs recovered from the WGS library of the photosynthetic picoeukaryotes fall into two different groups (CHIV3 and CHIV4 encode circovirus-like RC-Reps, whereas CHIV11 has a nanovirus-like protein), despite the fact that their CPs cluster together ( Fig. 4 ). Similarly, the CP of CHIV13 is closely related to the corresponding BSL_RDHV protein, but their RC-Reps group with geminiviruses and circoviruses, respectively ( Fig. 5 ). 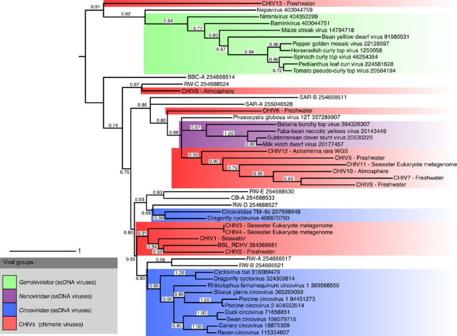Figure 5: Phylogenetic analysis of the CHIV RC-Reps. CHIVs are highlighted in red, circoviruses in blue, nanoviruses in purple and geminiviruses in green. Environmental sequences amplified from Reclaimed Water (RW), Chesapeake Bay (CB) or British Columbia (BBC) were taken as additional references24,34, as well asRC-Repgene from double-stranded DNA (dsDNA) algalPhaeocystis globosavirus 12T. Numbers at the branch points represent SH-like local support values (based on 1,000 resamples), and nodes with scores <0.5 were collapsed. NCBI GI numbers are indicated for all reference sequences. Table 1 RCR and S3H motifs of CHIV RC-Reps. Full size table Figure 5: Phylogenetic analysis of the CHIV RC-Reps. CHIVs are highlighted in red, circoviruses in blue, nanoviruses in purple and geminiviruses in green. Environmental sequences amplified from Reclaimed Water (RW), Chesapeake Bay (CB) or British Columbia (BBC) were taken as additional references [24] , [34] , as well as RC-Rep gene from double-stranded DNA (dsDNA) algal Phaeocystis globosa virus 12T. Numbers at the branch points represent SH-like local support values (based on 1,000 resamples), and nodes with scores <0.5 were collapsed. NCBI GI numbers are indicated for all reference sequences. Full size image Table 2 Statistical analysis of constrained trees. Full size table To compare the evolutionary patterns of CHIVs, circoviruses, nanoviruses, geminiviruses and tombusviruses, we have plotted the pairwise distances calculated for CPs from the representative members within each taxon against the corresponding distances between their replication proteins (Reps; Fig. 6a ). We found that in circoviruses, nanoviruses, geminiviruses and tombusviruses, the Reps are considerably less divergent that the corresponding CPs. Strikingly, the pattern is the opposite in CHIVs; RC-Reps are much more divergent than in any other virus taxon. In combination with the results of phylogenetic analysis ( Fig. 5 ), such sequence divergence of CHIV RC-Reps is most consistent with multiple independent events of RC-Rep gene replacement in different CHIVs. 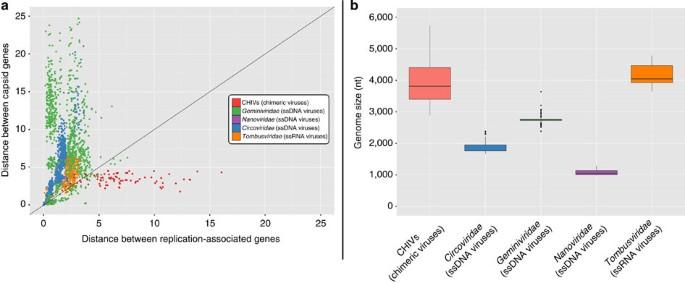Figure 6: Comparison of CHIVs with other ssDNA viruses and tombusviruses. (a) Evolutionary distance (Jones–Taylor–Thornton (JTT) model) for RC-Rep and CP sequences assessed between pairs of genomes within ssDNA and ssRNA families, and between CHIVs. (b) Box plot of genome size distribution in CHIVs (14 genomes), circoviruses (67), geminiviruses (464), nanoviruses (4) and tombusviruses (48). Whiskers correspond to the R ggplot library geom_boxplot function default paramers (for upper whisker: the highest value that is within 1.5*Inter-Quartile Range of the hinge, and for lower whisker: the smallest value that is within 1.5*Inter-Quartile Range of the hinge). Any value outside these whiskers is considered as an outlier and displayed as a dot. Figure 6: Comparison of CHIVs with other ssDNA viruses and tombusviruses. ( a ) Evolutionary distance (Jones–Taylor–Thornton (JTT) model) for RC-Rep and CP sequences assessed between pairs of genomes within ssDNA and ssRNA families, and between CHIVs. ( b ) Box plot of genome size distribution in CHIVs (14 genomes), circoviruses (67), geminiviruses (464), nanoviruses (4) and tombusviruses (48). Whiskers correspond to the R ggplot library geom_boxplot function default paramers (for upper whisker: the highest value that is within 1.5*Inter-Quartile Range of the hinge, and for lower whisker: the smallest value that is within 1.5*Inter-Quartile Range of the hinge). Any value outside these whiskers is considered as an outlier and displayed as a dot. Full size image Unicellular algae as recombination hotspots Although viromes studied here were assembled from a wide range of biomes ( Supplementary Data 1 ), CHIVs are exclusively retrieved from aquatic and atmospheric environments. Similarly, when microbial metagenomes are considered, CHIVs once again are identified only in aquatic samples. Three CHIV genomes (two of which are very similar, CHIV3 and CHIV4) are detected in two different samples enriched for the photosynthetic unicellular alga Bathycoccus , pointing towards potential association between algae and CHIVs. The fourth CHIV genome associated with aquatic microbes is found in the WGS library of A. rara . It is worth noting that foraminiferans are often engaged in endosymbiotic relationships and were found to host unicellular algae belonging to diverse lineages, including green algae, red algae, diatoms and dinoflagellates [47] . Consequently, it is possible that the CHIV contig associated with A. rara derives from an algal symbiont, rather than A. rara itself. At any rate, the association of different CHIV contigs with two different types of eukaryotes raises an intriguing possibility that unicellular eukaryotes serve as hosts for at least some CHIVs. Interestingly, we identified a close homologue (AET73220; E =4e−29, 35% identity) of CHIV12 RC-Rep (but not the CP) encoded in the genome of a giant double-stranded DNA virus, PgV-12T, infecting Phaeocystis globosa [48] , a photosynthetic unicellular algae. It has been recently demonstrated that satellite viruses and transposons integrate into the genome of the Lentille virus, a relative of mimiviruses [49] . It is tempting to speculate that ssDNA viruses and derived elements might represent a new class of molecular parasites preying on giant double-stranded DNA viruses. Regardless, the presence of the RC-Rep gene in the genome of PgV-12T lends additional support to the hypothesis that unicellular algae may host at least some of the CHIVs. More generally, parasitic and symbiotic relationships involving unicellular algae are highly prevalent in aquatic environments [50] and might be central for the emergence of new virus types, such as CHIVs, by providing a unique environment accessible for viruses infecting phylogenetically distant hosts. Such co-localization of various genetic elements of distinct origins and histories could also explain the evolutionary relationships between RC-Reps of prokaryotic plasmids and eukaryotic ssDNA viruses [12] , [13] , [15] , [21] , [22] . Recombination is known to have an important role in the evolution of eukaryotic ssDNA viruses [13] , [19] . However, interfamilial gene exchange has not been convincingly demonstrated for these viruses, suggesting that such recombination might be either uncommon or the recombinants are rarely retained in the population. In this light, pervasive exchange of RC-Rep genes in CHIVs is surprising. We hypothesize that the unusually frequent RC-Rep gene transfer in the CHIV lineage could have been instigated by incongruences between the capsid and RC-Rep proteins in the ancestral CHIV. It appears reasonable to assume that CP and RC-Rep, which evolved in the contexts of RNA and DNA viral genomes, respectively, would not immediately form a perfect match. Thus, RC-Rep genes could have been exchanged as long as the CP-Rep combination is not optimal. However, once the CP and the RC-Rep genes are sufficiently adapted to each other (that is, further ‘sampling’ decreases fitness) and/or viruses occupy a specific niche where ‘sampling’ is no longer possible, such high rate of gene exchange is expected to transit to a more conservative mode observed in other eukaryotic ssDNA viruses. Metagenomic studies have recently uncovered the unsuspected diversity of ssDNA viruses, many of which encode RC-Reps similar to those of geminiviruses, nanoviruses and, perhaps most commonly, circoviruses [17] , [18] . However, their CP genes are typically beyond recognition using sequence-based approaches, opening a possibility that these uncultured viruses represent highly divergent yet genuine members of the corresponding viral families. By contrast, CHIVs described here—despite being scattered throughout the RC-Rep phylogeny ( Fig. 5 )—all share a CP gene, which they apparently inherited from a common ancestor ( Fig. 4 ). Importantly, tombusvirus-like CP gene is not the only feature that distinguishes CHIVs from the three families of eukaryotic viruses mentioned above. CHIV genomes are also significantly larger than those of geminiviruses, nanoviruses and circoviruses, and are close in size to the ssRNA genomes of tombusviruses ( Fig. 6b ). Consequently, capsids larger than those of ssDNA viruses would be required to package such genomes. Interestingly, mechanical properties, such as persistence length, of ssRNA and ssDNA molecules are similar [51] , indicating that tombusvirus-like capsids would be well fitted to accommodate the larger genomes of CHIVs. Where do viruses with RNA virus-like capsids, DNA genomes and RC-Rep diversity spanning the major groups of eukaryotic ssDNA viruses fit in the virosphere? Obviously, CHIVs cannot be neatly placed into any one of the established groups of ssDNA viruses. Furthermore, evidence that RC-Rep genes can be exchanged between unrelated viruses blurs the borders between the major groups of eukaryotic ssDNA viruses and renders the RC-Rep-based classification of the uncultured ssDNA viruses into the circo-, nano- or gemini-like groups obsolete. Indeed, CHIVs with circovirus-like RC-Reps are as similar to circoviruses (that is, circovirus-like) [30] , as they are to tombusviruses [12] . Recognizing the limits of the RC-Rep-based approach in classifying uncultured ssDNA viruses, Rosario et al. [17] have recently proposed an alternative classification scheme based on a combination of various genomic properties of these viruses. According to the new scheme, viruses are categorized into eight groups (I–VIII) based on their genome orientation, the location of the intergenic region containing the potential stem loop structure, as well as the orientation of the nonanucleotide motif with respect to the RC-Rep gene [17] . The diversity of genome organizations observed in CHIVs spans six of the eight proposed groups ( Fig. 1 and Supplementary Data 2 ), suggesting that such classification scheme might not prove to be practical. More generally, none of the viral genes taken separately can adequately represent viral history [52] , especially so in the light of rampant horizontal gene exchange in the viral world [53] . Genetic mosaicism has been previously pointed out as a factor impeding meaningful classification of tailed bacteriophages (order Caudovirales) [54] . However, the coding capacity of tailed bacteriophages is typically large enough to accommodate a representative core gene set [55] , [56] sufficient for hierarchical clustering of these viruses into biologically significant subdivisions [57] , [58] . For viruses with small genomes, on the other hand, the effect of horizontal gene transfer on the ‘identity’ of a viral group is considerably more acute. Thus, eukaryotic ssDNA viruses, which usually encode only a handful of proteins, in our opinion, represent a clear-cut case of organisms for which ancient evolutionary history cannot be reconstructed employing whole-genome approaches. In a situation where objective means of virus classification are not applicable, a different—even if suboptimal—solution has to be sought. One way would be to classify CHIVs (and ssDNA viruses in general) based on their Reps into different viral groups, neglecting the history and nature of their CP genes. Such approach would be coherent with the Baltimore classification (that is, all viruses with ssDNA genomes would be collected together). However, such grouping would be inconsistent with our finding that RC-Reps were replaced on multiple occasions within the CHIV group. Furthermore, such scheme would be blind to the inferred structural uniformity of this viral group: all CHIVs are likely to possess similar capsids, considerably larger than those of ssDNA viruses but related in size and appearance to the capsids of tombus-like viruses ( Fig. 2 ). Notably, CPs are hallmarks of viruses and are less likely to leave the realm of virosphere than Reps that are often exchanged between unrelated viruses, plasmids and cellular chromosomes [59] . Thus, alternative approach would involve virus classification based on CPs. Which of these two classification schemes will prove to be more practical remains to be seen. Difficulties with classification of new ssDNA virus groups notwithstanding exploration of the viral world has presented valuable insights into the origin and evolution of viruses. It is now obvious that the virosphere is only gradually revealing its secrets—the more we sample the virosphere, the more unexpected connections we uncover between viruses that once were considered unrelated. Note added in proof: Following the revision of this article, Hewson et al . have described the identification of a new CHIV genome in samples collected from Oneida and Cayuga lakes (upstate New York, USA) [71] , further expanding our knowledge on the genetic diversity and environmental distribution of this peculiar group of chimeric viruses. Interestingly, the new ssDNA virus appears to be associated with planktonic crustaceans of the genus Daphnia . Genomic analysis showed that the new CHIV genome encodes a circovirus-like RC-Rep and displays an ambisense genome orientation, like in the case of CHIV3 and CHIV4, which are associated with seawater picoalga. Detection of CHIVs in assembled viromes A set of 103 published viromes available in public databases were downloaded and used in this study. These viromes were obtained from viral communities associated with different types of aquatic samples (freshwater, seawater and hypersaline ponds), eukaryote-associated flora (the human gut, saliva, lung, coral and fish), as well as with more peculiar biomes like microbialites or atmospheric samples ( Supplementary Data 1 ). All viromes were assembled with Newbler 2.6 (454 Life Sciences), with the following parameters: 98% similarity over 35 bp. A BLASTx search was computed to detect contigs containing genes similar to those of RNA viruses (extracted from the NCBI protein database on Aug 2012). Genes were predicted with MetaGeneAnnotator [60] for all contigs that were found to encode putative RNA virus capsid-like proteins (threshold of 50 on bitscore and 0.001 on e-value). Contigs containing at least two genes, one similar to an RNA virus capsid gene and one to the RC-Rep gene were considered as CHIVs ( Supplementary Data 1 ). All of these contigs presented coverage >7 × , and up to 395 × ( Supplementary Data 2 ). Screening of WGS libraries Different databases from the NCBI were screened for the presence of CHIVs based on the ten CPs from CHIVs (the nine contigs assembled in this study and the BSL_RDHV genome [30] ). Searches against genomic survey sequence, WGS and high-throughput genomic sequence libraries were performed using tBLASTn, whereas BLASTp was used to compare CHIV CP sequences to metagenomic proteins (env_nr). Putative CHIVs were detected in metagenomes targeting the small eukaryotic fraction in coastal upwelling waters off central Chile (NCBI GI:372349332 and 393314887) [37] . Reads from these two data sets were assembled with the same pipeline as the viromes, and three putative CHIV genomes were obtained. In addition, putative CHIV genome was retrieved from a WGS project of a foraminifera, Astrammina rara (NCBI Bioproject PRJNA47149; Contig ADNL01003178) [38] . Structural modelling and model quality assessment The three-dimensional model of the putative CP of CHIV10 was constructed using the advanced multi-template approach with MODELLER v9.9 (ref. 61 ). X-ray structures of tomato bushy stunt virus (TBSV; Protein Data Bank (PDB) ID: 2TBV), melon necrotic spot virus (MNSV; PDB ID: 2ZAH), carnation mottle virus (CMV; PDB ID: 1OPO) and turnip crinkle virus (TCV; PDB ID: 3ZXA) were used as templates. Sequence of CHIV10 CP was aligned with the corresponding sequences of TBSV, MNSV, CMV and TCV, and the resultant alignment was used to build a three-dimensional model of the putative CP of CHIV10. The initial model was optimized via multiple rounds of loop refinement with MODELLER. The stereochemical quality of the model was then assessed with ProSA-web [62] . ProSA-web quality ( Z ) score for the CHIV10 model was calculated to be −6.49, which is similar to the Z -scores determined for the template structures (TBSV, −5.18; MNSV, −6.26; CMV, −6.06; TCV, −3.39; Fig. 3 ). The MNSV virion map was downloaded from the VIPER database ( viperdb.scripps.edu/ ) and rendered using UCSF Chimera [63] . Phylogenetic analysis Multiple sequence alignments for RC-Rep and capsid genes were computed with MUSCLE [64] and manually curated (alignments are available from the authors upon request). Positions (560 and 289) were selected from the CP and RC-Rep alignments, respectively, and were used for subsequent phylogenetic analysis. Maximum-likelihood trees were calculated using FastTree [65] with Jones–Taylor–Thornton model of amino acid evolution and γ-CAT estimation of evolutionary rates across sites. Phylogenetic reconstructions with Bayesian MCMC (Markov chain Monte Carlo) yielded very similar tree topologies. The trees were annotated with Itol [66] . To test the monophyly of CHIV sequences in CP and Rep phylogenetic trees, two maximum-likelihood trees were computed for each alignment: one unconstrained and one with all CHIV sequences forced into a monophyletic group. TreeFinder [67] was used to compare the two topologies for each alignment through expected-likelihood weights and the approximately unbiased [68] test ( Table 2 ). Estimation of evolutionary distances between proteins MEGA 5 (ref. 69 ) was used to assess evolutionary distances between protein sequences of capsid and RC-Rep genes (Jones–Taylor–Thornton model, γ-parameter set to the default value of 1.3). For ssDNA and ssRNA viruses, all available genomes were downloaded from NCBI, and clustered based on taxonomy (one genome for each species) and on global sequence similarity (threshold of 75% identity) with Uclust [70] . Comparisons were made within each taxonomic group (Circoviridae, Geminiviridae, Nanoviridae and Tombusviridae ) and between CHIVs based on distinct multiple alignments computed with MUSCLE [64] . To keep the chart clear and viewable, only distances below 25 were taken, which removed 30 comparisons between Geminiviridae where RC-Rep protein distances were below 10 but capsid genes distances were between 25 and 100. The same set of sequences was used in the genome size box plot. Unclassified ssDNA and ssRNA viruses were not included in these analyses. Accession Codes: All CHIV genome sequences assembled in this study are available as annotated GenBank-formatted files through Dryad Digital Repository ( http://datadryad.org/pages/publicationBlackout ), doi: 10.5061/dryad.19m2k. How to cite this article: Roux, S. et al. Chimeric viruses blur the borders between the major groups of eukaryotic single-stranded DNA viruses. Nat. Commun. 4:2700 doi: 10.1038/ncomms3700 (2013).